The ARNT–STAT3 axis regulates the differentiation of intestinal intraepithelial TCRαβ+CD8αα+cells Intestinal intraepithelial T cells contribute to the regulation of inflammatory responses in the intestine; however, the molecular basis for their development and maintenance is unknown. The aryl hydrocarbon receptor complexes with the aryl hydrocarbon receptor nuclear translocator (ARNT) and senses environmental factors, including gut microbiota. Here, we identify ARNT as a critical regulator of the differentiation of TCRαβ + CD8αα + intestinal intraepithelial T cells. Mice deficient in either ARNT or aryl hydrocarbon receptor show a greater than- eight-fold reduction in the number of TCRαβ + CD8αα + intestinal intraepithelial T cells. The number of TCRαβ + CD8αα + intestinal intraepithelial T cells is increased by treatment with an aryl hydrocarbon receptor agonist in germ-free mice and is decreased by antibiotic treatment. The Arnt -deficient precursors of TCRαβ + CD8αα + intestinal intraepithelial T cells express low amounts of STAT3 and fail to differentiate towards the TCRαβ + CD8αα + cell fate after IL-15 stimulation, a deficiency that is overcome by overexpression of Stat3 . These data demonstrate that the ARNT–STAT3 axis is a critical regulator of TCRαβ + CD8αα + intestinal intraepithelial T-cell development and differentiation. The environment of the intestine includes a variety of microorganisms and foods. Various subsets of immune cells are located in the intestine, and they maintain immune tolerance by exerting competent immune reactions against pathogens [1] , [2] . T cells are located on both sides of the basement membrane of the intestinal epithelium. Among T cells, intraepithelial T cells (IELs) express either TCRγδ or TCRαβ. The CD4 − TCRαβ + IELs are divided into two subsets, one subset that expresses only CD8α and one subset that coexpresses CD8α and CD8β [2] . Although the function and origin of TCRαβ-positive CD8αα + IELs (TCRαβ + CD8αα + IELs) is poorly understood [3] , [4] , one study demonstrated that TCRαβ + CD8αα + IELs prevented colitis induced by the transfer of CD4 + CD45RB high T cells to SCID mice [3] . This result suggests that TCRαβ + CD8αα + IELs play a critical role in the regulatory function of the mucosal immune system. The aryl hydrocarbon receptor nuclear translocator (ARNT) is a transcriptional regulator [5] , [6] . ARNT belongs to the basic–helix–loop–helix–PAS protein family and functions as an essential dimerization partner with the aryl hydrocarbon receptor (AHR), and is involved in the hypoxia inducible factor-1α (HIF1α) signalling pathways [5] . Upon ligand binding, the AHR translocates to the nucleus and dimerizes with ARNT to form the AHR–ARNT heterodimer. Under hypoxic conditions, ARNT dimerizes with HIF1α, and the binding of this heterodimer to the Hif1a response element upregulates the transcription of genes, including several glycolytic enzymes [7] . Recent studies have revealed that AHR activation promotes Th17 differentiation with significant production of IL-22 (refs 8 , 9 , 10 ). We also demonstrated that Notch-stimulated CD4 + T cells upregulate IL-22 through AHR signalling [11] . Furthermore, one report demonstrated that AHR signalling controls TCRγδ + IELs by sensing dietary components [12] and showed that Ahr -deficient mice have a reduced number of TCRαβ + CD8αα + IELs [12] . However, it remains unclear as to the mechanism by which TCRαβ + CD8αα + IELs are regulated by environmental signals. Moreover, the molecular basis underlying AHR-mediated regulation of TCRαβ + CD8αα + IELs is not understood. Here, we show that Arnt -deficient mice possess approximately one-eighth the number of TCRαβ + CD8αα + IELs as wild-type mice. The precursors of TCRαβ + CD8αα + IELs express STAT3 at lower levels than control cells. Strikingly, the Stat3 -deficient mice have low numbers of TCRαβ + CD8αα + IELs. In the Arnt -deficient mice, overexpression of STAT3 in the TCRαβ + CD8αα + IEL precursors rescues the TCRαβ + CD8αα + IELs. These data indicate that the ARNT–STAT3 axis is critical for TCRαβ + CD8αα + IEL development, which suggests a unique interplay between the host immune system and the intestinal environment. Arnt -deficiency reduces the number of TCRαβ + CD8αα + IELs Arnt flox/flox mice were crossed with CD4- Cre transgenic (Arnt f/f -CD4) mice to delete Arnt from the T cells. The Arnt f/f -CD4 mice harboured six to eight times fewer TCRαβ + CD8αα + IELs compared with control CD4- Cre transgenic (Arnt +/+ -CD4) mice both in terms of frequencies ( Fig. 1a ) and absolute numbers ( Fig. 1b ). By contrast, compared with the controls, the Arnt f/f -CD4 mice had comparable levels of TCRαβ + CD8αβ + IELs both in terms of frequency ( Fig. 1a ) and absolute number ( Fig. 1b ). The development of TCRγδ + IELs was not impaired in the Arnt f/f -CD4 mice ( Fig. 1a ). Thy1.2 high TCRαβ + CD8αα + IELs lose Thy1.2 expression during differentiation [13] . More than 80% of the TCRαβ + CD8αα + IELs in the Arnt +/+ -CD4 mice were Thy1.2-negative, whereas approximately 70% of the TCRαβ + CD8αα + IELs in the Arnt f/f -CD4 mice highly expressed Thy1.2 ( Fig. 1a ). Furthermore, the Thy1.2-positive and Thy1.2-negative TCRαβ + CD8αα + IELs in the Arnt f/f -CD4 mice expressed granzyme B, an activation marker, at levels lower than those in the Arnt +/+ -CD4 mice ( Fig. 1c ). The majority of the TCRαβ + CD8αα + cells from both strains expressed CD69 ( Fig. 1c ). These data suggest that ARNT is important for the development or differentiation of TCRαβ + CD8αα + IELs in the small intestine. 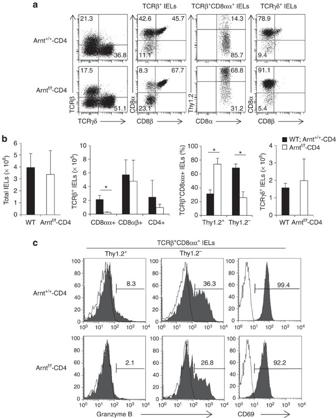Figure 1: Impairment of TCRαβ+CD8αα+IELs in Arntf/f-CD4 mice. (a) IELs from Arntf/f-CD4 and Arnt+/+-CD4 mice were stained with anti-TCRβ, TCRγ, CD4, CD8α, CD8β and Thy1.2 antibodies. The numbers in the dot plots indicate the percentages of cells represented in the quadrants. (b) The absolute numbers of the indicated IEL subsets in the individual mice were calculated from the relative percentage of each subset and the total IELs. The relative percentages of Thy1.2+or Thy1.2−cells in the TCRβ+CD8αα+cells are shown (n=5). Statistically significant differences: *P<0.05 (Studentt-test). The error bars indicate the means±s.d. (c) The expression of granzyme B or CD69 in the TCRαβ+CD8αα+IELs was evaluated by flow cytometry. The experiments in this figure represent the data from four independent experiments. Figure 1: Impairment of TCRαβ + CD8αα + IELs in Arnt f/f -CD4 mice. ( a ) IELs from Arnt f/f -CD4 and Arnt +/+ -CD4 mice were stained with anti-TCRβ, TCRγ, CD4, CD8α, CD8β and Thy1.2 antibodies. The numbers in the dot plots indicate the percentages of cells represented in the quadrants. ( b ) The absolute numbers of the indicated IEL subsets in the individual mice were calculated from the relative percentage of each subset and the total IELs. The relative percentages of Thy1.2 + or Thy1.2 − cells in the TCRβ + CD8αα + cells are shown ( n =5). Statistically significant differences: * P <0.05 (Student t -test). The error bars indicate the means±s.d. ( c ) The expression of granzyme B or CD69 in the TCRαβ + CD8αα + IELs was evaluated by flow cytometry. The experiments in this figure represent the data from four independent experiments. Full size image ARNT in CD8 + cells regulates TCRαβ + CD8αα + IELs TCRαβ + CD8αα + IELs are derived from CD4 − CD8 − TCRαβ + cells in the thymus [2] . To identify the cell types in which Arnt was deleted by the CD4- Cre transgene, we crossed Arnt +/+ -CD4 or Arnt f/f -CD4 mice with CAG–CAT–GFP (Arnt +/+ -CD4-CAG or Arnt f/f -CD4-CAG, respectively) mice in which GFP expression was directed upon Cre-mediated excision of the loxP-flanked chloramphenicol acetyltransferase (CAT) gene located between the CAG promoter and the GFP gene [14] . Approximately 90% of the CD4 + or CD4 − CD8 − TCRαβ + cells in the thymus expressed GFP in the Arnt +/+ -CD4-CAG mice and Arnt f/f -CD4-CAG mice ( Fig. 2a ). In contrast, 10–20% of the CD4 − CD8 − TCRβ − cells were positive for GFP in the Arnt +/+ -CD4-CAG and Arnt f/f -CD4-CAG mice ( Fig. 2a ). Approximately 90% of the TCRαβ + CD8αα + IELs in either the Arnt +/+ -CD4-CAG or Arnt f/f -CD4-CAG mice expressed GFP, whereas GFP was barely detected in the TCRγδ + IELs from the Arnt f/f -CD4-CAG mice ( Fig. 2a ). These data demonstrate that the CD4- Cre transgene deleted Arnt at a precursor stage of the TCRαβ + CD8αα + IELs in the thymus but not in the TCRγδ + lineage of IELs. 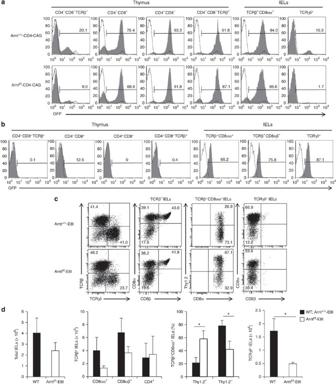Figure 2: Impairment of TCRαβ+CD8αα+IELs in Arntf/f-E8I mice. (a) Thymocytes or IELs from Arntf/f-CD4-CAG and Arnt+/+-CD4-CAG mice were stained with anti-CD4, -CD8α, -CD8β, -TCRγ or -TCRβ antibody, and the GFP-positive cells were evaluated by flow cytometry. Line: Arnt+/+mice, Shadow: Arntf/f-CD4-CAG or Arnt+/+-CD4-CAG mice. (b) The expression of GFP in the TCRαβ+CD8αα+IELs from the Arnt+/+-E81 mice was evaluated by flow cytometry. Line: Arnt+/+mice, Shadow: Arnt+/+-E81 mice. (c) IELs from Arntf/f-E8I and Arnt+/+-E8I mice were stained with anti-TCRβ, TCRγ, CD4, CD8α, CD8β and Thy1.2 antibodies. The numbers in the dot plots indicate the percentages of cells represented in the quadrants. (d) The absolute numbers of the indicated IEL subsets in the individual mice were calculated from the relative percentage of each subset and the total IELs (n=5). Statistically significant differences: *P<0.05 (Student’st-test). The error bars indicate the means±s.d. The experiments in this figure represent the data from four independent experiments. Figure 2: Impairment of TCRαβ + CD8αα + IELs in Arnt f/f -E8I mice. ( a ) Thymocytes or IELs from Arnt f/f -CD4-CAG and Arnt +/+ -CD4-CAG mice were stained with anti-CD4, -CD8α, -CD8β, -TCRγ or -TCRβ antibody, and the GFP-positive cells were evaluated by flow cytometry. Line: Arnt +/+ mice, Shadow: Arnt f/f -CD4-CAG or Arnt +/+ -CD4-CAG mice. ( b ) The expression of GFP in the TCRαβ + CD8αα + IELs from the Arnt +/+ -E81 mice was evaluated by flow cytometry. Line: Arnt +/+ mice, Shadow: Arnt +/+ -E81 mice. ( c ) IELs from Arnt f/f -E8I and Arnt +/+ -E8I mice were stained with anti-TCRβ, TCRγ, CD4, CD8α, CD8β and Thy1.2 antibodies. The numbers in the dot plots indicate the percentages of cells represented in the quadrants. ( d ) The absolute numbers of the indicated IEL subsets in the individual mice were calculated from the relative percentage of each subset and the total IELs ( n =5). Statistically significant differences: * P <0.05 (Student’s t -test). The error bars indicate the means±s.d. The experiments in this figure represent the data from four independent experiments. Full size image To better understand the roles of ARNT in the development and/or differentiation of TCRαβ + CD8αα + IELs, Arnt flox/flox or Arnt +/+ mice were crossed with E81- Cre transgenic (Arnt f/f -E81 or Arnt +/+ -E81, respectively) mice in which the expression of the Cre–GFP fusion protein was directed by E8I (ref. 15 ). GFP was expressed in the TCRαβ + CD8αα + IELs, TCRαβ + CD8αβ + IELs and TCRγδ + IELs but not in the CD4 − CD8 − TCRβ + cells in the thymus of the Arnt +/+ -E81 mice ( Fig. 2b ). Therefore, the E8I- Cre transgene deletes Arnt at a mature stage of the TCRαβ + CD8αα + IELs rather than at an immature CD4 − CD8 − TCRβ + cell stage in the thymus. The Arnt f/f -E81 mice have similar numbers of TCRαβ + CD8αα + and TCRαβ + CD8αβ + cells compared with the Arnt +/+ -E81 mice, but reduced numbers of TCRγδ + IELs compared with the Arnt +/+ -E81 mice ( Fig. 2c ). However, the percentage of Thy1.2 + cells in the TCRαβ + CD8αα + IELs from the Arnt f/f -E81 mice was greater than that from Arnt +/+ -E8I mice ( Fig. 2c ), indicating that deletion of Arnt at a mature stage impaired the differentiation of TCRαβ + CD8αα + IELs in the small intestine. Taken together, the data demonstrate that ARNT is critical for the differentiation of TCRαβ + CD8αα + IELs at both the immature and mature stages, and that ARNT plays an important role in the development or survival of TCRγδ + IELs. Ahr - but not Hif1a -deficiency reduces TCRαβ + CD8αα + IELs ARNT can form a complex with either AHR or HIF1α [5] . Therefore, we determined whether a deficiency in either Ahr or Hif1a affected the differentiation of TCRαβ + CD8αα + IELs. Hif1a flox/flox or Hif1a +/+ mice were crossed with the CD4-Cre transgenic mice (Hif1α f/f -CD4 or Hif1α +/+ -CD4, respectively). The Hif1α f/f -CD4 mice had comparable numbers of TCRαβ + CD8αα + , TCRαβ + CD8αβ + and TCRγδ + IELs relative to the control mice ( Fig. 3a ). The percentages of Thy1.2 + cells in the TCRαβ + CD8αα + IELs were also similar in the Hif1α f/f -CD4 and control mice ( Fig. 3a ). By contrast, Ahr- deficient ( Ahr −/− ) mice showed reduced numbers of TCRαβ + CD8αα + IELs, and the number of Thy1.2 + cells in the TCRαβ + CD8αα + IELs was higher in the Ahr −/− mice than the Ahr +/− mice ( Fig. 3b ). These data indicate that Arnt/Ahr but not Arnt/HIF1α is critical for the development of TCRαβ + CD8αα + IELs. 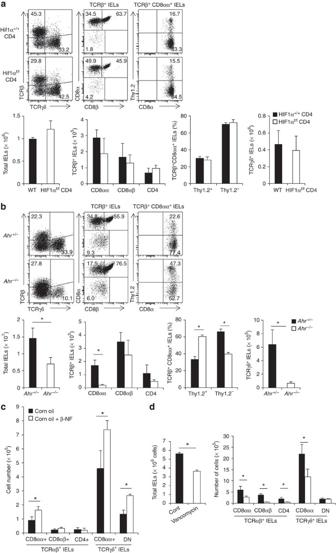Figure 3:Ahr-deficiency impairs the development of TCRαβ+CD8αα+IELs. IELs from (a) Hif1αf/f-CD4 and Hif1α+/+-CD4 mice or (b)Ahr+/+andAhr−/−mice were stained with anti-CD4, -CD8α, -CD8β, -TCRβ and -TCRγ antibodies. The numbers in the dot plots indicate the percentages of cells represented in the quadrants. The total number of cells in each of the indicated populations was counted (n=5). (c) Germ-free mice were treated with oral β-NF (1 mg per mouse, every day for three weeks). The absolute numbers of the indicated IEL subsets in the individual mice were calculated from the relative percentage of each subset and the total IELs (n=5; DN; CD4−CD8−). (d) C57BL/6 mice were treated with vancomycin administered in the drinking water (1 g l−1) for 3 weeks. The absolute numbers of the indicated IEL subsets in the individual mice were calculated from the relative percentage of each subset and the total IELs (n=5). Statistically significant differences: *P<0.05 (Student’st-test). Error bars indicate the means±s.d. The experiments in this figure represent the data from four independent experiments. Figure 3: Ahr- deficiency impairs the development of TCRαβ + CD8αα + IELs. IELs from ( a ) Hif1α f/f -CD4 and Hif1α +/+ -CD4 mice or ( b ) Ahr +/+ and Ahr −/− mice were stained with anti-CD4, -CD8α, -CD8β, -TCRβ and -TCRγ antibodies. The numbers in the dot plots indicate the percentages of cells represented in the quadrants. The total number of cells in each of the indicated populations was counted ( n =5). ( c ) Germ-free mice were treated with oral β-NF (1 mg per mouse, every day for three weeks). The absolute numbers of the indicated IEL subsets in the individual mice were calculated from the relative percentage of each subset and the total IELs ( n =5; DN; CD4 − CD8 − ). ( d ) C57BL/6 mice were treated with vancomycin administered in the drinking water (1 g l −1 ) for 3 weeks. The absolute numbers of the indicated IEL subsets in the individual mice were calculated from the relative percentage of each subset and the total IELs ( n =5). Statistically significant differences: * P <0.05 (Student’s t -test). Error bars indicate the means±s.d. The experiments in this figure represent the data from four independent experiments. Full size image A previous study demonstrated that germ-free mice have lower numbers of total IELs and TCRαβ + CD8αα + IELs than mice under specific pathogen-free conditions [16] . To determine whether microbiota are associated with the ARNT/AHR-mediated differentiation of IELs, the AHR agonist β-naphthoflavone (β-NF) was orally administered to germ-free mice. The administration of β-NF increased the total number of TCRαβ + CD8αα + IELs together with the TCRγδ + IELs but not the TCRαβ + CD8αβ + IELs ( Fig. 3c ), indicating that AHR signalling is critical for the development of TCRαβ + CD8αα + IELs. We then administered vancomycin to mice housed under SPF conditions to determine which bacteria contributed to TCRαβ + CD8αα + IEL differentiation. The administration of vancomycin to C57BL/6 mice reduced the total number of IELs, and three populations of TCRαβ + IELs and TCRγδ + IELs ( Fig. 3d ). These data indicate that vancomycin-sensitive bacteria are involved in the differentiation of IELs, including TCRαβ + CD8αα + IELs. Arnt -deficiency in T cells does not affect IEL precursors Next, we determined whether the putative IEL precursor population, CD4 − CD8 − TCRβ + NK1.1 − B220 − CD5 + cells [17] , was reduced in Arnt f/f -CD4 mice. The total thymocytes and CD4 − CD8 − TCRβ + NK1.1 − B220 − CD5 + cells in the thymus were present at similar frequencies ( Fig. 4a ) and absolute numbers ( Fig. 4b ) in the Arnt f/f -CD4 and control mice. 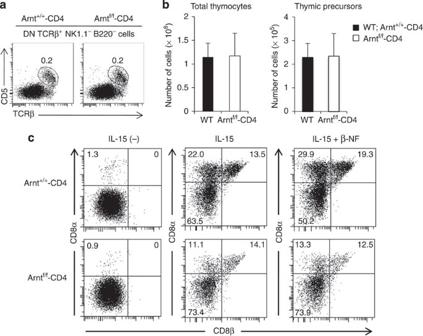Figure 4:Arnt-deficiency in T cells does not affect the development of IEL precursors. (a) Thymocytes from Arntf/f-CD4 and Arnt+/+-CD4 mice were stained with antibodies against CD4, CD8, B220, TCRβ, NK1.1 and CD5. Cells expressing TCRβ and CD5 but not CD4, CD8, B220 or NK1.1 were evaluated. The numbers in the dot plots indicate the percentages of CD4−CD8−B220−NK1.1−CD5+TCRβ+cells. (b) The absolute number of CD4−CD8−B220−NK1.1−CD5+TCRβ+cells in the thymus of Arntf/f-CD4 and Arnt+/+-CD4 mice was counted (n=10). The error bars indicate the means±s.d. (c) CD4−CD8−B220−NK1.1−CD5+TCRβ+cells in the thymus of Arnt+/+-CD4 mice were stimulated with β-NF (50 nM)for 7 days, after which the cells were stained with antibodies against TCRβ, CD8α and CD8β, and evaluated by flow cytometry. The numbers in the dot plots indicate the percentages of cells represented in the quadrants. The experiments in this figure represent the data from four independent experiments. Figure 4: Arnt -deficiency in T cells does not affect the development of IEL precursors. ( a ) Thymocytes from Arnt f/f -CD4 and Arnt +/+ -CD4 mice were stained with antibodies against CD4, CD8, B220, TCRβ, NK1.1 and CD5. Cells expressing TCRβ and CD5 but not CD4, CD8, B220 or NK1.1 were evaluated. The numbers in the dot plots indicate the percentages of CD4 − CD8 − B220 − NK1.1 − CD5 + TCRβ + cells. ( b ) The absolute number of CD4 − CD8 − B220 − NK1.1 − CD5 + TCRβ + cells in the thymus of Arnt f/f -CD4 and Arnt +/+ -CD4 mice was counted ( n =10). The error bars indicate the means±s.d. ( c ) CD4 − CD8 − B220 − NK1.1 − CD5 + TCRβ + cells in the thymus of Arnt +/+ -CD4 mice were stimulated with β-NF (50 n M) for 7 days, after which the cells were stained with antibodies against TCRβ, CD8α and CD8β, and evaluated by flow cytometry. The numbers in the dot plots indicate the percentages of cells represented in the quadrants. The experiments in this figure represent the data from four independent experiments. Full size image IL-15 is a critical cytokine for the development of IELs [13] , [18] , [19] . Previous studies indicated that treatment of CD4 − CD8 − TCRβ + NK1.1 − B220 − CD5 + cells with IL-15 increased the expression of CD8αα [19] , [20] . Consistent with these previous reports, IL-15-mediated stimulation of CD4 − CD8 − TCRβ + NK1.1 − B220 − CD5 + cells from control mice increased the expression of CD8αα ( Fig. 4c ). In contrast, Arnt- deficiency in this population decreased the IL-15-mediated increase in the expression of CD8αα ( Fig. 4c ), suggesting that Arnt -deficiency is associated with the IL-15 signalling pathway. Using this experimental system, we next evaluated whether ARNT- or AHR-signalling contributed to further differentiation of CD4 − CD8 − TCRβ + NK1.1 − B220 − CD5 + cells. Therefore, we stimulated the CD4 − CD8 − TCRβ + NK1.1 − B220 − CD5 + population with β-NF. Stimulation of the CD4 − CD8 − TCRβ + NK1.1 − B220 − CD5 + cells from the Arnt +/+ -CD4 mice with β-NF increased the number of TCRαβ + CD8αα + cells, whereas β-NF did not increase the number of TCRαβ + CD8αα + cells from the Arnt f/f -CD4 mice ( Fig. 4c ). These data suggest that ARNT is critical for the differentiation of TCRαβ + CD8αα + IELs from precursors to a mature stage rather than the development of the precursors of TCRαβ + CD8αα + IELs. STAT5 is not involved in Arnt-mediated IEL development To examine the association between ARNT and IL-15, we used Arnt f/f -CD4 mice to analyse the expression patterns of the IL-15α receptor, CD122 and CD132 (common γ-chain) that constitute the functional IL-15 receptor in TCRαβ + CD8αα + IELs. The expression levels of these three receptors were similar in the Arnt f/f -CD4 mice and control mice ( Fig. 5a ). STAT5 is a downstream signalling molecule for IL-15 (ref. 21 ). We sought to determine whether overexpression of constitutively active Stat5 driven by the CD2 promoter could rescue the development of TCRαβ + CD8αα + IELs in the Arnt f/f -CD4 mice. The Arnt +/+ -CD4 mice crossed with the constitutively active Stat5 transgenic (Arnt +/+ -CD4 Stat5-CA) mice exhibited increased development of the total TCRαβ + IELs and TCRαβ + CD8αα + IELs ( Fig. 5b ). In contrast, the overexpression of constitutively active Stat5 in the Arnt f/f -CD4 (Arnt f/f -CD4 Stat5-CA) mice did not increase the development of TCRαβ + CD8αα + IELs ( Fig. 5b ). Furthermore, the constitutively active Stat5 did not promote the differentiation of Thy1.2 − TCRαβ + CD8αα + IELs from Thy1.2 + TCRαβ + CD8αα + IELs in the Arnt f/f -CD4 mice ( Fig. 5b ). These data indicate that Stat5 is not involved in the ARNT-mediated development of TCRαβ + CD8αα + IELs. 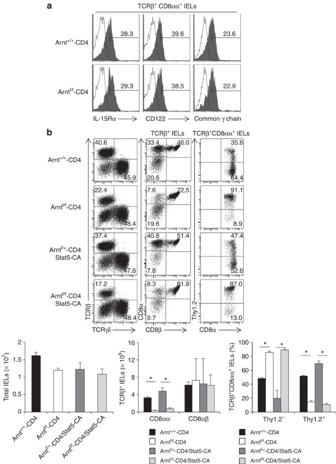Figure 5: STAT5 is not involved in ARNT-mediated IEL development. (a) TCRβ+CD8αα+IELs were stained with anti-IL-15Rα, -CD122, and common γ-chain antibodies, and the antigen expression was evaluated by flow cytometry. The number indicates the percentage of positive cells for each molecule. (b) Arntf/f-CD4 and Arnt+/+-CD4 mice were crossed with constitutively activeStat5and the IELs were stained with antibodies against CD4, CD8α, CD8β, TCRβ, TCRγ and Thy1.2. The cells were analysed by flow cytometry. The numbers in the dot plots indicate the percentages of cells represented in the quadrants. The total number of cells in each of the indicated populations was counted (n=5). Statistically significant differences: *P<0.05 (Student’st-test). The error bars indicate the means±s.d. The experiments in this figure represent the data from four independent experiments. Figure 5: STAT5 is not involved in ARNT-mediated IEL development. ( a ) TCRβ + CD8αα + IELs were stained with anti-IL-15Rα, -CD122, and common γ-chain antibodies, and the antigen expression was evaluated by flow cytometry. The number indicates the percentage of positive cells for each molecule. ( b ) Arnt f/f -CD4 and Arnt +/+ -CD4 mice were crossed with constitutively active Stat5 and the IELs were stained with antibodies against CD4, CD8α, CD8β, TCRβ, TCRγ and Thy1.2. The cells were analysed by flow cytometry. The numbers in the dot plots indicate the percentages of cells represented in the quadrants. The total number of cells in each of the indicated populations was counted ( n =5). Statistically significant differences: * P <0.05 (Student’s t -test). The error bars indicate the means±s.d. The experiments in this figure represent the data from four independent experiments. Full size image Stat3 -deficiency reduces TCRαβ + CD8αα + IEL development STAT3 is another downstream signalling molecule for the IL-15 receptor [21] . We compared the expression levels of STAT3 in CD4 − CD8 − TCRβ + NK1.1 − B220 − CD5 + cells from the Arnt f/f -CD4 and Arnt +/+ -CD4 mice ( Fig. 6a ). The proportion of STAT3-positive cells and the STAT3 intensity in CD4 − CD8 − TCRβ + NK1.1 − B220 − CD5 + cells from the Arnt f/f -CD4 mice were lower than those in the Arnt +/+ -CD4 mice, whereas the expression of STAT3 was comparable in the mature CD4 + T cells in the spleens ( Fig. 6a ). However, the expression of the Stat3 mRNA was comparable in the CD4 − CD8 − TCRβ + NK1.1 − B220 − CD5 + cells from the Arnt +/+ -CD4 and Arnt f/f -CD4 mice ( Fig. 6b ). 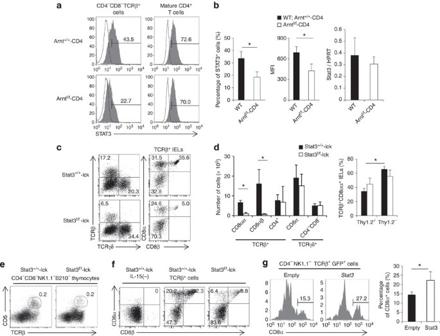Figure 6:Stat3-deficiency impairs the development of TCRαβ+CD8αα+IELs. The expression of STAT3 in CD4−CD8−B220−NK1.1−CD5+TCRβ+cells from Arntf/f-CD4 and Arnt+/+-CD4 mice was evaluated by flow cytometry. (a) The number in each histogram indicates the percentage of STAT3-positive cells in the CD4−CD8−B220−NK1.1−CD5+TCRβ+population. (b) The number of STAT3-positive cells and the mean fluorescence intensity or mRNA level of STAT3 in CD4−CD8−B220−NK1.1−CD5+TCRβ+cells was evaluated in Arntf/f-CD4 and Arnt+/+-CD4 mice (n=5). (c) IELs from Stat3f/f-lck and Stat3+/+-lck mice were stained with anti-CD4, -CD8α, -CD8β, -TCRβ and -TCRγ antibodies. The numbers in the dot plots indicate the percentages of cells represented in the quadrants. (d) IELs from the Stat3f/f-lck and Stat3+/+-lck mice were stained with anti-CD4, -CD8α, -CD8β, -Thy1.2, -TCRβ and -TCRγ antibodies, and the number of each population in the TCRβ+or TCRγ+cells was counted. (e) Thymocytes from the Stat3f/f-lck and Stat3+/+-lck mice were stained with antibodies against CD4, CD8, B220, TCRβ, NK1.1 and CD5. The cells positive for the expression of TCRβ and CD5 and negative for CD4, CD8, B220 and NK1.1 were evaluated. The numbers in the dot plots indicate the percentages of CD4−CD8−B220−NK1.1−CD5+TCRβ+cells. (f) CD4−CD8−TCRβ+NK1.1−B220−CD5+cells from Stat3f/f-lck and Stat3+/+-lck mice were cultured in the presence of IL-15 (100 ng ml−1). Seven days later, the cells were stained with antibodies against TCRβ, CD8α and CD8β and evaluated by flow cytometry. The numbers in the dot plots indicate the percentages of cells represented in the quadrants. (g) CD4−CD8−TCRβ+NK1.1−B220−CD5+cells from Arntf/f-CD4 and Arnt+/+-CD4 mice were transduced withStat3in the presence of IL-15 (100 ng ml−1). Seven days later, the cells were stained with antibodies against TCRβ, CD8α and CD8β and evaluated by flow cytometry. The numbers in the dot plots indicate the percentages of cells represented in the quadrants. The percentage of CD8α+cells was counted in four independent experiments. Statistically significant differences: *P<0.05 (Student’st-test). The error bars indicate the means±s.d. The experiments in this figure represent the data from four independent experiments. Figure 6: Stat3 -deficiency impairs the development of TCRαβ + CD8αα + IELs. The expression of STAT3 in CD4 − CD8 − B220 − NK1.1 − CD5 + TCRβ + cells from Arnt f/f -CD4 and Arnt +/+ -CD4 mice was evaluated by flow cytometry. ( a ) The number in each histogram indicates the percentage of STAT3-positive cells in the CD4 − CD8 − B220 − NK1.1 − CD5 + TCRβ + population. ( b ) The number of STAT3-positive cells and the mean fluorescence intensity or mRNA level of STAT3 in CD4 − CD8 − B220 − NK1.1 − CD5 + TCRβ + cells was evaluated in Arnt f/f -CD4 and Arnt +/+ -CD4 mice ( n =5). ( c ) IELs from Stat3 f/f -lck and Stat3 +/+ -lck mice were stained with anti-CD4, -CD8α, -CD8β, -TCRβ and -TCRγ antibodies. The numbers in the dot plots indicate the percentages of cells represented in the quadrants. ( d ) IELs from the Stat3 f/f -lck and Stat3 +/+ -lck mice were stained with anti-CD4, -CD8α, -CD8β, -Thy1.2, -TCRβ and -TCRγ antibodies, and the number of each population in the TCRβ + or TCRγ + cells was counted. ( e ) Thymocytes from the Stat3 f/f -lck and Stat3 +/+ -lck mice were stained with antibodies against CD4, CD8, B220, TCRβ, NK1.1 and CD5. The cells positive for the expression of TCRβ and CD5 and negative for CD4, CD8, B220 and NK1.1 were evaluated. The numbers in the dot plots indicate the percentages of CD4 − CD8 − B220 − NK1.1 − CD5 + TCRβ + cells. ( f ) CD4 − CD8 − TCRβ + NK1.1 − B220 − CD5 + cells from Stat3 f/f -lck and Stat3 +/+ -lck mice were cultured in the presence of IL-15 (100 ng ml −1 ). Seven days later, the cells were stained with antibodies against TCRβ, CD8α and CD8β and evaluated by flow cytometry. The numbers in the dot plots indicate the percentages of cells represented in the quadrants. ( g ) CD4 − CD8 − TCRβ + NK1.1 − B220 − CD5 + cells from Arnt f/f -CD4 and Arnt +/+ -CD4 mice were transduced with Stat3 in the presence of IL-15 (100 ng ml −1 ). Seven days later, the cells were stained with antibodies against TCRβ, CD8α and CD8β and evaluated by flow cytometry. The numbers in the dot plots indicate the percentages of cells represented in the quadrants. The percentage of CD8α + cells was counted in four independent experiments. Statistically significant differences: * P <0.05 (Student’s t -test). The error bars indicate the means±s.d. The experiments in this figure represent the data from four independent experiments. Full size image To determine the contribution of STAT3 to the development of TCRαβ + CD8αα + IELs, we first evaluated the development of TCRαβ + CD8αα + IELs in Stat3 flox/flox or Stat3 +/+ mice crossed with lck- Cre transgenic (Stat3 f/f -lck or Stat3 +/+ -lck, respectively) mice. The Stat3 f/f -lck mice showed an approximately five-fold reduction in TCRαβ + CD8αα + and TCRαβ + CD8αβ + IELs but had comparable numbers of TCRαβ + CD4 + and TCRγδ + IELs relative to the control mice ( Fig. 6c ). Although the Thy1.2 − population was larger than the Thy1.2 + population in the control TCRαβ + CD8αα + IELs, the ratios of the populations were fairly similar in Stat3 -deficient TCRαβ + CD8αα + IELs ( Fig. 6d ). These data indicate that STAT3 selectively controls the development of TCRαβ + CD8αα + and TCRαβ + CD8αβ + IELs and also regulates the differentiation of TCRαβ + CD8αα + cells. The Stat3 f/f -lck mice had a comparable number of CD4 − CD8 − TCRβ + NK1.1 − B220 − CD5 + cells in the thymus compared with the control mice ( Fig. 6e ). Cultures of CD4 − CD8 − TCRβ + NK1.1 − B220 − CD5 + cells from the Stat3 f/f -lck mice in the presence of IL-15 failed to give rise to CD8αα + cells in contrast to the increased differentiation of CD8αα + cells from the Stat3 +/+ -lck mice ( Fig. 6f ). Furthermore, stimulation of the CD4 − CD8 − TCRβ + NK1.1 − B220 − CD5 + cells from the Stat3 f/f -lck mice with β-NF did not increase the number of TCRαβ + CD8αα + IELs ( Supplementary Fig. S1 ). Finally, we sought to determine whether the impaired development of TCRαβ + CD8αα + IELs due to Arnt -deficiency was caused by low STAT3 expression in the precursor population. Therefore, we transduced Stat3 into the CD4 − CD8 − TCRβ + NK1.1 − B220 − CD5 + cells from the Arnt f/f -CD4 mice and stimulated the cells with IL-15 for 7 days. The overexpression of Stat3 in the CD4 − CD8 − TCRβ + NK1.1 − B220 − CD5 + cells from the Arnt f/f -CD4 mice increased the number of CD8αα + cells compared with the control virus-infected cells ( Fig. 6g ). Taken together, those data indicate that ARNT-mediated upregulation of STAT3 is critical for the development of TCRαβ + CD8αα + IELs. A variety of environmental molecules interact with the host, particularly in the intestine. One of the molecules that sense environmental stimuli is the AHR [5] . Recent studies have demonstrated that AHR is a master regulator of drug metabolism and that it controls cell growth and differentiation through the recognition of endogenous ligands [5] , [22] . Here, we demonstrate that ARNT/AHR is critical for the development of TCRαβ + CD8αα + IELs, most probably by sensing commensal bacteria. This finding contrasts with the critical role of AHR in TCRγδ + IEL development by sensing dietary components [12] . Notably, ARNT regulates the expression of STAT3, a downstream molecule for the IL-15 receptor. We found that deletion of Stat3 during the early stages of thymocyte maturation reduced the development of TCRαβ + CD8αα + IELs, whereas overexpression of Stat3 in Arnt -deficient cells rescued the development of TCRαβ + CD8αα + IELs. This newly identified molecular network indicates a unique interplay between the host immune system and environmental signals in the intestine. IL-15 is critical for the development of TCRαβ + CD8αα + IELs [18] , [19] . The role of IL-15 in the development of TCRαβ + CD8αα + IELs was suggested by the observation that IL-15 could support the expression of CD8α by the precursors of TCRαβ + CD8αα + IELs in vitro [19] , [20] , [23] . Here, we demonstrate that IL-15 failed to cause the expression of CD8α in the precursors of Arnt -deficient TCRαβ + CD8αα + IELs due to low expression of Stat3 . Overexpression of Stat3 in Arnt -deficient TCRαβ + CD8αα + IEL precursors rescued the differentiation of TCRαβ + CD8αα + IELs. The IL-15 receptor utilizes several signalling molecules, including STAT3 and STAT5 (ref. 21 ). However, overexpression of constitutively active Stat5 in Arnt -deficient cells did not rescue the development of TCRαβ + CD8αα + IELs. These data indicate that ARNT signalling controls Stat3 expression in IEL precursors, which contributes to IL-15-mediated development of TCRαβ + CD8αα + IELs. Therefore, the ARNT–STAT3 axis may control lineage-specific genetic programs required for the development of TCRαβ + CD8αα + IELs, although one study showed that IL-15 was important for the survival of IELs [19] . As to the mechanism by which ARNT regulates the expression of Stat3 , Stat3 expression in the mature CD4 + T cells in the spleens of Arnt f/f -CD4 mice was not reduced. This observation suggests that ARNT-mediated regulation of Stat3 occurs in a T-cell-type- or maturation-specific manner. For the molecular mechanism of ARNT-mediated regulation of Stat3 , our data indicate that Arnt -deficiency does not affect Stat3 mRNA expression. These data suggest that ARNT controls Stat3 gene expression post-transcriptionally. We provide evidence that ARNT is involved in Stat3 gene expression related to IL-15-mediated development of TCRαβ + CD8αα + IELs. However, it remains possible that either IL-15 or ARNT have independent roles in the development of TCRαβ + CD8αα + IELs. This issue should be investigated by comparing the development of TCRαβ + CD8αα + IELs in IL-15- and Arnt- double-deficient mice and single gene deficient mice. Furthermore, because STAT3 is required for signalling through other cytokine receptors, it would be interesting to determine the association of TCRαβ + CD8αα + IEL development with other cytokines that utilize STAT3 as a signalling molecule. We found that when Arnt was deleted from E81- Cre transgene mice, the number of TCRαβ + CD8αα + IELs was not significantly reduced, whereas their maturation was inhibited as determined by Thy1.2 expression. These data suggest that ARNT signalling is required not only during the precursor stage of TCRαβ + CD8αα + IELs but also during final maturation in the small intestine. For TCRγδ + IELs, a previous study postulated that AHR signalling induced by dietary components is important for the maintenance of TCRγδ + IELs [12] , which also suggests that AHR/ARNT regulates the maintenance of TCRγδ + IELs. Although the number of TCRγδ + IELs in the Arnt f/f -E81 mice is reduced, the Arnt f/f -CD4 mice have similar numbers of TCRγδ + IELs compared to control mice. Similar to previous studies that have suggested that TCRγδ + IELs are not derived from the CD4 + CD8 + stage in the thymus [2] , the low expression of GFP in the TCRγδ + IELs from the Arnt f/f -CD4-CAG mice also suggests that TCRγδ + IELs are not derived from the CD4 + CD8 + stage. Ideally, the association between the ARNT/AHR and commensal bacteria, and their role in TCRαβ + CD8αα + IEL development should be analysed in germ-free Ahr- or Arnt -deficient mice. Nonetheless, the data presented here show that the administration of an AHR agonist in germ-free mice increased the number of TCRαβ + CD8αα + IELs. This result suggests that commensal bacteria stimulate AHR signalling leading to the development of TCRαβ + CD8αα + IELs. We also demonstrated that the treatment of mice with vancomycin under SPF conditions, which primarily eradicated Gram-positive bacteria, reduced the number of TCRαβ + CD8αα + IELs, although it is unclear whether the microbiota directly provide AHR ligands or indirectly contribute to the production of AHR ligands from host cells. A previous study has shown that dietary components stimulate AHR, a process that is involved in the development of TCRγδ + IELs [12] . Therefore, various environmental signals should regulate the development or differentiation of IELs. Currently, there is little understanding of the advantage gained by bacteria in promoting the development of IELs, including TCRαβ + CD8αα + IELs. A proposed role for TCRαβ + CD8αα + IELs is to eliminate transformed or injured epithelial cells [2] . Thus, it is possible that the proper development of TCRαβ + CD8αα + IELs by bacteria may contribute to the health of the epithelial layer that supports the commensal bacteria. Because TCRαβ + CD8αα + IELs play a protective role in intestinal inflammation [3] , our data suggest that AHR stimulation may have a role in suppressing inflammatory bowel diseases by stimulating TCRαβ + CD8αα + IELs. Indeed, previous studies have demonstrated that AHR agonist treatment suppresses DSS-mediated intestinal inflammatory responses [24] , [25] , [26] . Conversely, the inhibition of STAT3 by antagonists may have adverse effects on intestinal homoeostasis, although STAT3 is considered a target molecule for the treatment of both cancer [27] and psoriasis [28] . Therefore, further studies are required to determine whether modulation of the ARNT–STAT3 axis in a time- or tissue-specific manner has clinical therapeutic potential. Mice Six- to eight-week-old C57BL/6 mice were purchased from Japan SLC (Hamamatsu, Japan). The Arnt flox/flox mice [29] were crossed with CD4- Cre mice, the Arnt flox/flox mice were crossed with E8I- Cre mice [15] , the Hif1α flox/flox mice [30] were crossed with CD4- Cre mice and the Stat3 flox/flox mice [31] were crossed with Lck- Cre mice . Constitutively active Stat5 transgenic mice [32] (provided by Dr M. Farrar, University of Minnesota, MN), CAG–CAT–GFP mice [14] (provided from Dr J. Miyazaki), and Ahr -deficient mice [33] were maintained under specific pathogen-free conditions in the animal research centre at the University of Tokushima, Japan. Germ-free BALB/c mice were purchased from CLEA Japan (Tokyo, Japan) and were housed in flexible vinyl isolators. These mice were provided sterilized water and sterilized commercial CL-2 pellets (CLEA Japan). Female mice were used for all experiments. All experiments were performed in accordance with institutional guidelines for animal care at the University of Tokushima. Flow cytometry Fluorochrome-conjugated monoclonal antibodies specific for mouse CD8α (25-0081-81), CD5 (11-0051-81), IL-15Rα (12-7149-80), CD122 (12-1221-81) and anti-mouse IgG (11-4011-85) were purchased from eBioscience (San Diego, CA, USA). Antibodies specific for CD4 (552051), CD69 (557392), common γ-chain (18362D), B220 (558108) and CD8β (550798) were obtained from BD Biosciences (San Jose, CA, USA). Antibodies specific for TCRβ (109208), NK1.1 (108710), TCRγ (118116) and streptavidin-PE (405204) were purchased from Biolegend (San Diego, CA, USA). Antibodies for granzyme B (MHGB05) and mouse IgG (MHG05) were purchased from Life Technologies (Grand Island, NY, USA), and an antibody for STAT3 (9139) was purchased from Cell Signaling Technologies (Danvers, MA, USA). All samples were resuspended in PBS staining buffer containing 2% FCS and 0.01% NaN 3 and preincubated for 15 min at 4 °C with 2.4G2 supernatant to block the Fc receptor. The samples were then washed and stained with the specific mAb (1:100 dilution) for 20 min at 4 °C. For intracellular staining, the cells were fixed with 4% paraformaldehyde and permeabilized with 0.01% saponin-containing buffer. The data were collected on a FACS CantoII flow cytometer (BD Biosciences, San Jose, CA, USA) and analysed using either FACS Diva (BD Biosciences) or FlowJo (Tree Star, OR, USA) software. Isolation of intraepithelial lymphocytes Small intestines were removed and cleaned of mesentery, the Peyer’s patches were removed and the intestines were opened longitudinally. The intestines were sectioned into 1-cm pieces and washed twice in cold PBS. The pieces were stirred at 37 °C for 20 min in RPMI 1640 medium containing 5% FCS, 20 mM HEPES, 25 mM NaHCO 3 , 100 μg ml −1 penicillin/streptomycin and 1 mM EDTA. The IELs in the supernatant were collected at the interface of 40/75% Percoll gradients. Administration of β-naphthoflavone to mice β-NF was purchased from Wako Pure Chemicals (Tokyo, Japan). One milligram per mouse β-NF or corn oil was orally administered to germ-free mice every day for three weeks. Antibiotics treatment C57BL/6 mice, 6–7 weeks old, were treated with vancomycin (1 g l −1 ) administered in the drinking water for 3 weeks. Real-time PCR The total RNA was extracted with TRIzol (Life Technologies) or RNeasy Plus Micro Kits (Qiagen, Valencia, CA, USA), and the cDNA was synthesized using the Omniscript RT Kit (Qiagen) after digestion of the genomic DNA with DNase (Promega, Madison, WI, USA). Gene expression was analysed using the SYBR Premix Ex Taq II (TAKARA, Otsu, Shiga, Japan) and primers using an ABI7500 real time PCR system (Applied Biosystems, Foster City, CA). The following primers were used: STAT3, forward 5′-TGCCCATGGCTACCTGTT-3′ and reverse 5′-GAACCTCCTGGGCTTAGTCC-3′; and HPRT, forward 5′-AGCCTAAGATGAGCGCAAGT-3′ and reverse 5′-TTACTAGGCAGATGGCCAC-3′ In vitro cell culture CD4 − CD8 − TCRβ + B220 − NK1.1 − thymocytes were enriched using a cell sorter and cultured in 24-well plates (1 × 10 5 cells). Recombinant murine IL-15 (Biolegend; 100 ng ml −1 ) and/or β-NF (50 nM) (Wako Chemicals) was added on day zero and the cells were analysed on day 7. Cell sorting was performed using a FACS AriaIII Flow Cytometer (BD biosciences). The cDNA of murine Stat3 was cloned into a pKE004 retroviral vector [34] . The retroviruses were constructed by transfecting vectors into plat-E cells [35] (provided by Dr T. Kitamura, Tokyo University). The thymocytes were infected with retrovirus once on the first day of the cell culture. Statistical analysis For all experiments, the significance of differences between groups was calculated using the Mann–Whitney U -test for unpaired data. The differences were considered significant when P <0.05. How to cite this article: Nakajima, K. et al . The ARNT–STAT3 axis regulates the differentiation of intestinal intraepithelial TCRαβ + CD8αα + cells. Nat. Commun. 4:2112 doi: 10.1038/ncomms3112 (2013).